Genomic insights into salt adaptation in a desert poplar Despite the high economic and ecological importance of forests, our knowledge of the genomic evolution of trees under salt stress remains very limited. Here we report the genome sequence of the desert poplar, Populus euphratica , which exhibits high tolerance to salt stress. Its genome is very similar and collinear to that of the closely related mesophytic congener, P. trichocarpa . However, we find that several gene families likely to be involved in tolerance to salt stress contain significantly more gene copies within the P. euphratica lineage. Furthermore, genes showing evidence of positive selection are significantly enriched in functional categories related to salt stress. Some of these genes, and others within the same categories, are significantly upregulated under salt stress relative to their expression in another salt-sensitive poplar. Our results provide an important background for understanding tree adaptation to salt stress and facilitating the genetic improvement of cultivated poplars for saline soils. Forests dominate much of the terrestrial landscape [1] . However, forest trees rarely occur on saline soils and little is known of the genetic basis of their tolerance to salt stress despite strong demand for their cultivation on highly saline soils in many parts of the world [2] . Members of the genus Populus are used as a model forest species for diverse studies not only because of their amenability to experimental and genetic manipulation, but also because of their high economic and ecological importance as the most widely cultivated tree throughout the northern hemisphere [3] , [4] . More than 30 wild Populus species occur across diverse habitats over a wide geographical range, thereby providing an excellent system for unravelling the genetic bases of adaptive divergence [4] . Populus euphratica Oliv., which is native to desert regions ranging from western China to North Africa, is characterized by extraordinary adaptation to salt stress [5] , [6] , [7] , [8] . Notably, at high salinity it maintains higher growth and photosynthetic rates than other poplar species [9] , [10] and can survive concentrations of NaCl in nutrient solution up to 450 mM [11] . In this study, we examine genomic differences between a xeric desert poplar and its mesophytic congener, P. trichocarpa , for which a high-quality reference genome is available [12] . We further examine gene expression differences following salt stress treatment in a comparison with another salt-sensitive congener, P. tomentosa . Our comparisons highlight the genetic bases of salt tolerance in the desert poplar. Genome sequencing and assembly Because of the limitations of next-generation sequencing for complex genome assembly [13] and the high levels of polymorphism found in this non-domesticated and open-pollinated species ( Supplementary Fig. 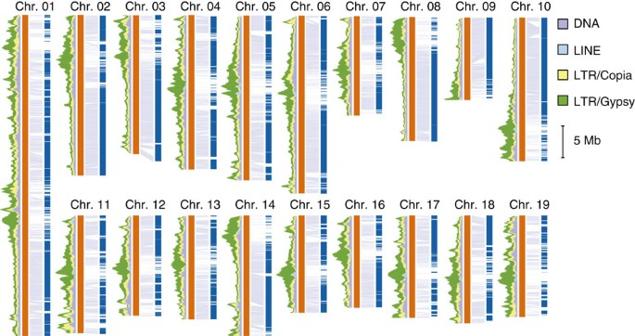Figure 1: Collinearity between theP. euphraticaandP. trichocarpagenomes. TheP. euphraticascaffolds (blue) inferred to be collinear are linked (grey lines) toP. trichocarpachromosomes (orange). The proportion of the repeat elements (left) across the chromosomes is indicated for 400 kb sliding windows at 50 kb steps. DNA transposable elements are shown in purple, long interspersed elements (LINE) are shown in light blue, Copia and Gypsy elements of LTR retrotransposons are shown in yellow and green, respectively. S1 ), we employed a newly developed fosmid-pooling strategy [14] to sequence and assemble the P. euphratica genome ( Table 1 and Supplementary Methods ). Hierarchical assembly using 67.1 Gb (~112 × ) whole-genome shotgun reads ( Supplementary Table S1 ), combined with more than 200 × high-quality reads from 66,240 fosmid clones ( Supplementary Table S2 ), yielded a final assembly with a total length of 496.5 Mb ( Supplementary Table S3 ), representing 83.7% of the P. euphratica nucleotide space ( Supplementary Tables S4 and S5 ). The contig N50 of the assembled sequence was 40.4 Kb (longest, 728.4 Kb) and scaffold N50 was 482 Kb (longest, 8.8 Mb; Table 1 ), which were comparable to those of other plant genome assemblies generated by next-generation sequencing technology ( Supplementary Table S6 ). Sequencing depth distribution showed that over 92.5% of the assembly was covered by more than 20 × ( Supplementary Figs S2 and S3 ), ensuring a high single-base accuracy. The heterozygosity level in P. euphratica was ~0.5% ( Supplementary Tables S7 and S8 , and Supplementary Fig. S4 ), which is almost twice that in P. trichocarpa (0.26%) [12] . The assembly covered 97.3% of the 516,712 Populus expressed sequence tags ( Supplementary Table S9 ) and 97.7% of the 7 complete fosmids sequenced by Sanger sequencing ( Supplementary Table S10 and Supplementary Fig. S5 ), without any obvious misassembly occurring. The coverage of the core eukaryotic genes was estimated to be 94.35% for the P. euphratica assembly ( Supplementary Table S11 ), which is comparable to the estimate for P. trichocarpa (93.95%). All of these statistics supported that our draft genome sequence has high contiguity, coverage and accuracy, further demonstrating the feasibility of this hierarchical approach for de novo sequencing and assembly of a complex genome with high heterozygosity [14] . Table 1 Statistics for the assembly of the Populus euphratica genome. Full size table Genome annotation Using a combination of homology-based searches and de novo annotation, we found that ~44% of the P. euphratica genome is composed of repetitive elements ( Supplementary Table S12 ), similar to that of the P. trichocarpa genome (47%; Fig. 1 ). Long-terminal repeats (LTRs) were the most abundant repeat class, representing 36.7% and 33.1% of the P. euphratica and P. trichocarpa genomes, respectively ( Supplementary Table S13 ). The distribution of repeat divergence rates revealed a peak of gypsy LTR at 11% in P. euphratica ( Supplementary Fig. S6 ), which is likely to reflect a relatively recent expansion of this LTR family in the P. euphratica lineage. Figure 1: Collinearity between the P. euphratica and P. trichocarpa genomes. The P. euphratica scaffolds (blue) inferred to be collinear are linked (grey lines) to P. trichocarpa chromosomes (orange). The proportion of the repeat elements (left) across the chromosomes is indicated for 400 kb sliding windows at 50 kb steps. DNA transposable elements are shown in purple, long interspersed elements (LINE) are shown in light blue, Copia and Gypsy elements of LTR retrotransposons are shown in yellow and green, respectively. Full size image A total of 34,279 protein-coding genes were predicted to be present in the P. euphratica genome ( Supplementary Table S14 and Supplementary Fig. S7 ), 96.6% of which were supported by expressed sequence tags and/or homology-based searching with only 3.4% derived solely from de novo gene predictions ( Supplementary Fig. S8 ). Functional annotation confirmed that 94.3% of the predicted genes had known homologues in protein databases ( Supplementary Table S15 ). Small RNA sequencing data supported the occurrence of 152 conserved and 114 candidate novel microRNAs predicted from the P. euphratica genome ( Supplementary Table S16 , Supplementary Data 1 and 2 , and Supplementary Figs S9–S11 ), most of which were extensively up/downregulated in response to salt stress ( Supplementary Table S17 and Supplementary Fig. S12 ). In addition, we also identified 764 transfer RNAs, 706 ribosomal RNAs and 4,826 small nuclear RNAs ( Supplementary Table S18 ). Genome evolution In accordance with previous research [12] , [15] , the distribution of the fourfold degenerate synonymous sites of the third codons (4DTv) value between duplicated genes showed similar peaks (~0.09 and ~0.59) in both P. euphratica and P. trichocarpa genomes, suggesting that two ancient whole-genome duplication (WGD) events had occurred in the Populus lineage ( Supplementary Table S19 , Supplementary Figs S13 and S14 ). These shared WGDs were also confirmed by the extensive collinearity between the genomes of both species ( Fig. 1 ). A total of 1,214 collinear blocks >10 kb in length, corresponding to 323 Mb (65% of the assembly) and 332 Mb (76%) in the P. euphratica and P. trichocarpa genomes, respectively, were identified ( Supplementary Table S20 ). Assuming that the recent WGD occurred around 65 million years ago (Mya) [12] , divergence between P. euphratica and P. trichocarpa can be placed to ~14 Mya (4DTv, ~0.02), which approximates to that estimated from phylogenetic analysis (~8 Mya; Supplementary Fig. S15 ). We identified and designed a total of 18,938 universal pairs of simple sequence repeat primers in the collinear regions, which can be converted into genetic markers across most poplar species ( Supplementary Data 3 and Supplementary Table S21 ). These simple sequence repeat markers, as well as the intraspecific or interspecific nucleotide variation in collinear regions, will facilitate genetic dissection of agronomically important traits and accelerate the genetic improvement of cultivated poplars, particularly for growth on saline soils. Adaptation to a saline environment Copy number within gene families has been reported to vary greatly between closely related, divergent species [16] , [17] . Both gene family and InterProScan domain analysis revealed that several gene families related to salt stress were substantially expanded in P. euphratica compared with other plant species ( Fig. 2a , Supplementary Tables S22–S24 , and Supplementary Figs S16 and S17 ). For example, the HKT1 (high-affinity K + transporter 1) gene family, which encodes Na + /K + transporters that have important roles in affecting or determining salt tolerance in plants [18] , expanded from one member in the P. trichocarpa genome to four in the P. euphratica genome. Three of these genes occurred as tandem duplicates in P. euphratica , which together corresponded to a HKT1- like pseudogene in P. trichocarpa ( Fig. 2b ). HKT1 transporters have a key role in limiting Na + transport from roots to shoots in Arabidopsis [19] , and may account for the lower rate of ion uptake and transport recorded in P. euphratica [9] , [20] , [21] . The gene family encoding P-type H + -ATPases also had more copies in the P. euphratica genome than in the P. trichocarpa genome ( Fig. 2c ). These P-type ATPases provide the basic energy for Na + /H + antiporters by sustaining an electrochemical H + gradient across the plasma membrane, thus making an important contribution to maintenance of low Na + concentrations in P. euphratica [22] , [23] . Other expanded gene families include those encoding antioxidative enzymes [24] , such as CAT (catalase) and GR1 (glutathione reductase), and genes involved in abscisic acid (ABA) signalling regulation [25] , such as GCR2 (G-protein-coupled receptor 2) and PLD (phospholipase D). Heat-shock proteins usually protect cells against salinity by controlling the proper folding and conformation of proteins [26] . Several of these families (for example, HSP20 , HSP70 and HSP90 ) were expanded in the P. euphratica genome. In addition, the P. euphratica genome has more copies of BADH (betaine aldehyde dehydrogenase) and GolS4 (galactinol synthase 4), which encode key enzymes involved in biosynthesis of critical solutes that have roles in osmotic adjustment pathways under salt stress [27] , [28] . 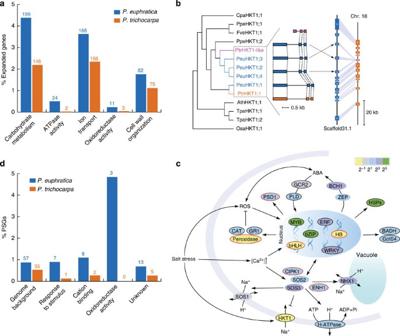Figure 2: Adaptation ofP. euphraticato salt stress. (a) Comparison of the proportions of expanded genes in theP. euphraticaandP. trichocarpalineages relative to their common ancestor. The number of expanded genes of each class is indicated above each bar. (b) Tandem duplications ofHKT1genes. Note that thePtrHKT1-like gene is pseudogenized inP. trichocarpa. (c) PSGs and expanded key genes in salt-stress response pathways ofP. euphratica. Boxes with borders indicate PSGs (red) and expanded (black)P. euphraticagenes, and the filled colors correspond to their degree of regulation in FPKMtreatment/FPKMcontrolin response to salt stress. (d) Comparison of the proportions of PSGs in theP. euphraticaandP. trichocarpalineages. The number of PSGs of each class is indicated above each bar. FPKM, fragments per kilobase of exon per million fragments mapped. Figure 2: Adaptation of P. euphratica to salt stress. ( a ) Comparison of the proportions of expanded genes in the P. euphratica and P. trichocarpa lineages relative to their common ancestor. The number of expanded genes of each class is indicated above each bar. ( b ) Tandem duplications of HKT1 genes. Note that the PtrHKT1- like gene is pseudogenized in P. trichocarpa . ( c ) PSGs and expanded key genes in salt-stress response pathways of P. euphratica . Boxes with borders indicate PSGs (red) and expanded (black) P. euphratica genes, and the filled colors correspond to their degree of regulation in FPKM treatment /FPKM control in response to salt stress. ( d ) Comparison of the proportions of PSGs in the P. euphratica and P. trichocarpa lineages. The number of PSGs of each class is indicated above each bar. FPKM, fragments per kilobase of exon per million fragments mapped. Full size image Adaptive divergence at the molecular level may also be reflected by an increased rate of non-synonymous changes within genes involved in adaptation [29] . In collinear regions, we identified 18,262 high-confidence 1:1 orthologous genes between P. euphratica and P. trichocarpa , with a mean protein similarity close to 98.94% ( Supplementary Fig. S18 ). The genes with elevated pairwise genetic differentiation were primarily enriched in ‘photosynthetic electron transport chain’, ‘heat acclimation’, ‘oxidoreductase activity’ and ‘cation channel activity’ ( Supplementary Table S25 ), indicating rapid evolution and/or adaptive divergence in these functions between P. euphratica and P. trichocarpa . Of the 6,545 high-confidence orthologues identified among 10 plant species ( Supplementary Fig. S16 ), we detected 57 positively selected genes (PSGs) in the P. euphratica lineage ( Supplementary Table S26 ), which is significantly greater than the number (35 PSGs) in the P. trichocarpa lineage ( P -value=0.014 by the Fisher’s exact test). Compared with P. trichocarpa PSGs, P. euphratica PSGs were significantly enriched ( P -value ≤0.05 by the Fisher’s exact test) in ‘response to stimulus’, ‘cation binding’ and ‘oxidoreductase activity’ ( Fig. 2d ). They included ENH1 (enhancer of sos3-1 ), which encodes a chloroplast-localized rubredoxin-like protein and has an important role in mediation of both ion homeostasis and reactive oxygen species detoxification [30] ; CIPK1 (CBL-interacting protein kinase 1), a protein kinase interacting strongly with the calcium sensors CBL1 and CBL9, and alternatively controlling ABA-dependent and ABA-independent stress responses in Arabidopsis [31] ; and PSD1 (phosphatidylserine decarboxylase 1) encoding a crucial enzyme catalysing production of phosphatidylethanolamine and therefore raising stress tolerance by increasing the flexibility of cell membranes [32] ( Fig. 2c ). Several genes encoding transcription factors such as HB40, bHLH87 and AP2/ERF, and oxidoreductases such as peroxidase, 2-oxoglutarate and Fe(II)-dependent oxygenase, also showed signs of positive selection. To examine the genome-wide responses to salt stress of this desert poplar, we performed a series of deep transcriptome sequencings ( Supplementary Table S27 ) that identified 6,727, 3,954 and 3,733 genes that were differentially expressed in salt-stressed calluses, leaves and roots of seedlings, respectively ( Supplementary Data 4–6 and Supplementary Fig. S19 ). These differentially expressed genes (DEGs), which included those comprising expanded gene families and also those bearing the signature of positive selection ( Fig. 2c , Supplementary Table S28 , and Supplementary Figs S20 and S21 ), were similarly enriched in functional categories, such as ‘oxidoreductase activity’, ‘transcription factor activity’ and ‘ion transport’ ( Fig. 3a ). Several expanded gene families in the P . euphratica genome comprised transcription factors ( Supplementary Table S24 ), for example, Myb , ERF , bZIP and WRKY , having a role in the regulation of gene expression in response to abiotic stress [33] . Some of these were extensively upregulated in response to salt stress ( Fig. 2c ; Supplementary Tables S28 and S29 ). Furthermore, the key genes regulating Na + /H + antiporters and controlling ion homeostasis [34] ( Supplementary Table S30 ), for example, NHX1 (Na + /H + exchanger 1), SOS2 (salt overly sensitive 2) and SOS3 , and those involved in the biosynthesis of ABA [35] , [36] , for example, BCH1 (β-carotene hydroxylase 1) and ZEP (zeaxanthin epoxidase), were upregulated in salt-stressed samples, which is consistent with previous research [37] . 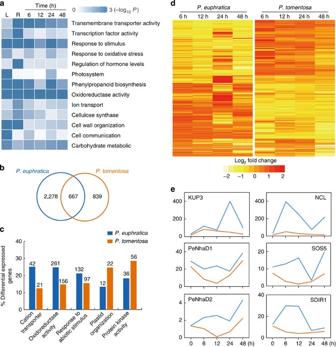Figure 3: Comparative transcriptomics ofP. euphraticaandP. tomentosaunder salt stress. (a) Functional category enrichment (P-value ≤0.05 by the Fisher's exact test) of DEGs inP. euphraticaleaves (L), roots (R) and time-course profiles. (b) Venn diagram of the number of DEGs inP. euphraticaandP. tomentosaunder salt stress (Supplementary Methods). (c) DEGs proportions inP. euphraticaandP. tomentosa. The number of DEGs of each class is indicated above each bar. (d) Expression of the DEGs identified inP. euphraticaand/orP. tomentosa. The heatmap was generated from hierarchical cluster analysis of genes. (e) Transcript levels of the genes showing different expression patterns betweenP. euphratica(blue) andP. tomentosa(orange). The transcript levels were determined by fragments per kilobase of exon per million fragments mapped (FPKM). Figure 3: Comparative transcriptomics of P. euphratica and P. tomentosa under salt stress. ( a ) Functional category enrichment ( P -value ≤0.05 by the Fisher's exact test) of DEGs in P. euphratica leaves (L), roots (R) and time-course profiles. ( b ) Venn diagram of the number of DEGs in P. euphratica and P. tomentosa under salt stress ( Supplementary Methods ). ( c ) DEGs proportions in P. euphratica and P. tomentosa . The number of DEGs of each class is indicated above each bar. ( d ) Expression of the DEGs identified in P. euphratica and/or P. tomentosa . The heatmap was generated from hierarchical cluster analysis of genes. ( e ) Transcript levels of the genes showing different expression patterns between P. euphratica (blue) and P. tomentosa (orange). The transcript levels were determined by fragments per kilobase of exon per million fragments mapped (FPKM). Full size image We further compared the expression profiles of the P. euphratica calluses in response to salt stress with those of the P. tomentosa (a salt-sensitive poplar [21] ) calluses ( Supplementary Table S31 , Supplementary Figs S22 and S23 ). The results showed that many of the DEGs (2,278) were specific to P. euphratica ( Fig 3b ), and that more genes involved in ‘cation transporter’, ‘oxidoreductase activity’ and ‘response to abiotic stimulus’ were induced in P. euphratica than in P. tomentosa ( Fig. 3c ). Clustering analysis suggested that many of the DEGs exhibited different regulatory patterns in response to salinity between these two species ( Fig. 3d ). For example, the K + uptake transporter KUP3 was extensively upregulated after 24 h of salt stress in P. euphratica , but was maintained at control levels in P. tomentosa ( Fig. 3e ), indicating a critical role of this gene in controlling K + homeostasis in P. euphratica . Transcript levels of this gene are strongly induced by K + starvation in Arabidopsis [38] . Previous research suggested that PeNhaD1 , encoding a NhaD-type Na + /H + antiporter, has a role in mediating sodium tolerance in P. euphratica [39] . Consistent with this, we identified two gene members encoding NhaD-type antiporters, both of which maintained transcript levels in P. euphratica , but which significantly reduced transcript levels under salt stress after 12 h in P. tomentosa before regaining control levels after 24 h ( Fig. 3e ). Another transporter encoding gene, NCL (Na + /Ca 2+ exchanger-like protein), involved in the maintenance of Ca 2+ homeostasis under salt stress in Arabidopsis [40] , was strongly upregulated in P. euphratica relative to its expression in salt-sensitive P. tomentosa . In addition, SOS5 , a gene encoding a putative cell surface adhesion protein for the maintenance of cell wall integrity and architecture under salt stress in Arabidopsis [41] , was downregulated in P. tomentosa after 12 h of salt stress, in contrast to maintenance of transcript levels recorded in P. euphratica . We further found that the gene SDIR1 (salt-and drought-induced ring finger 1), whose overexpression improves drought tolerance in transgenic rice [42] , was specifically upregulated after 6 h and maintained high transcript levels until 12 h after salt stress in P. euphratica . Finally, transcription factors, such as ERF3 and NAC042 , and the oxidoreductases AOX1D (alternative oxidase 1D) and NDA2 (alternative NAD(P)H dehydrogenase 2), exhibited different expression patterns under salt stress in P. euphratica relative to those recorded in P. tomentosa ( Supplementary Fig. S24 ). Abiotic stress factors, especially salinity and drought, restrict plant biomass production and pose an increasing threat to sustainable agriculture and forestry worldwide. Numerous studies have been conducted on the genetic and molecular mechanisms underlying salt tolerance in plants [18] , [19] , [30] , [31] , and have included genomic analyses of the extremophiles Thellungiella parvula [16] and T. salsuginea [43] . However, our current understanding of these aspects of salt tolerance remains limited, especially for woody plants [22] , [27] . Populus euphratica is an excellent candidate for the analysis of salt tolerance [22] , as it displays apoplastic sodium accumulation and develops leaf succulence after prolonged salt exposure [8] . Consequently, in the last decade it has become a model for elucidating both physiological and molecular mechanisms of salt tolerance in tree species [5] , [6] , [7] , [8] , [9] , [10] , [11] . Using a newly developed fosmid-pooling strategy [14] , we sequenced and assembled the complex genome of P. euphratica with high heterozygosity and compared it with the closely related salt-sensitive model plant, P. trichocarpa . We found that P. euphratica diverged from P. trichocarpa within the last 8 to 14 million years ( Supplementary Fig. S15 ). Although both species shared at least two WGDs and exhibited extensive collinearity across the gene space ( Fig. 1 and Supplementary Fig. S13 ), species-specific genes involved in stress tolerance, such as ‘ion transport’, ‘ATPase activity’, ‘transcript factor activity’ and ‘oxidoreductase activity’, were selectively expanded and/or positively selected in the P. euphratica genome ( Fig. 2 and Supplementary Tables S23–S26 ). In this regard, the Na + /K + transporter HKT1 is of particular interest, because it is similarly expanded as tandem duplicated copies in both T. parvula [16] and T. salsuginea [43] . Further functional analysis of this gene family is needed to understand its critical role in salt tolerance in plants. In addition, other genes involved in ion transport and homeostasis, such as NhaD1 , KUP3 and NCL , were distinctly upregulated under salt stress when compared with another salt-sensitive poplar, P. tomentosa . Our analyses taken together suggest that P. euphratica may have increased its salt tolerance through duplication and/or upregulation of multiple genes involved in ion transport and homeostasis. These findings are important for an improved understanding of tree adaptation to salt stress and for accelerating the genetic improvement of cultivated poplars for growth on saline soils. Genome sequencing and assembly Genomic DNA was extracted from callus induced from P. euphratica shoots. Paired-end and mate-pair Illumina libraries were constructed with multiple insert sizes (138–40 kb) according to the manufacturer’s instructions. In addition, 66,240 fosmid clones with 40 kb in length were randomly selected and two small insert (250 and 500 bp) libraries were constructed for each clone. All libraries were sequenced on the Illumina Genome Analyzer and HiSeq 2000 sequencing system. The raw reads were processed by removing low-quality reads, adapter sequences and possible contaminated reads. Then a hierarchical strategy [14] was used for genome assembly ( Supplementary Methods ). Gene prediction We used the homology-based and de novo methods, as well as RNA-seq data, to predict genes in the P. euphratica genome. For homology-based gene prediction, protein sequences from five plants ( P. trichocarpa , Ricinus communis , Prunus persica , Cucumis sativus and Glycine max ) were initially mapped onto the P. euphratica genome using TBLASTN and the homologous genome sequences were aligned against the matching proteins using GeneWise [44] for accurate spliced alignments. Next, we used the de novo gene prediction methods Augustus [45] and GenScan [46] to predict protein-coding genes, using parameters trained for P. euphratica and A. thaliana . We then integrated the homologues and those from de novo approaches using GLEAN [47] to produce a consensus gene set. In addition, we aligned all the RNA-seq reads to the reference genome by TopHat [48] , assembled the transcripts using Cufflinks [49] and predicted the open reading frames from the resultant data. Finally, we combined the GLEAN set with the gene models produced from RNA-seq to generate a more confident gene set. Collinear block and genome duplication identification Pairwise whole-genome alignment between P. euphratica and P. trichocarpa was constructed using the BLAST algorithm, and the scaffolds of P. euphratica were anchored to the P. trichocarpa corresponding chromosomes based on the consensus order of matched regions. To detect the signature of genome duplication, the programme MCSCAN [50] was used to define a duplicated block. At least five genes are required to call synteny. For each duplicated block, the 4DTv values were calculated and distributions were plotted. Gene family clusters The protein-coding genes from nine plant species ( P. trichocarpa , Ricinus communis , Arabidopsis thaliana , Thellungiella parvula , Carica papaya , Fragaria vesca , Prunus persica , Vitis vinifera and Oryza sativa ) were downloaded. The longest translation form was chosen to represent each gene, and stretches of genes encoding fewer than 50 amino acids were filtered out. The OrthoMCL [51] method was then used to cluster all the genes into paralogous and orthologous groups. The 1,776 single-copy gene families obtained from this analysis were used to reconstruct phylogenies and estimate divergence time using MrBayes [52] and the MCMCtree programme implemented in the Phylogenetic Analysis by Maximum Likelihood [53] . Calibration times were obtained from the TimeTree database ( http://www.timetree.org/ ). Identification of PSGs Using the orthologues identified by OrthoMCL as a raw data set, we first masked sites with low quality ( phred -like quality score<20) and that were detected as single nucleotide variants in P. euphratica coding sequences. We then aligned them using the codon option in the Probabilistic Alignment Kit [54] programme for the detection of positive selection. Alignments shorter than 150 bp after removing sites with ambiguous data were discarded. Finally, we obtained 6,545 high-confidence orthologues within the two poplar species and at least three of the other eight species ( R. communis , A. thaliana , T. parvula , C. papaya , F. vesca , P. persica , V. vinifera and O. sativa ), averaging ~7.7 species per gene. These alignments together with an unrooted phylogenetic tree (constructed as described above) were used for subsequent molecular evolutionary analysis. For the estimation of the lineage-specific evolutionary rate, the values of K a , K s and K a / K s were calculated for 10,000 concatenated alignments constructed from 150 randomly chosen genes using the Codeml programme with the free-ratio model in the Phylogenetic Analysis by Maximum Likelihood [53] package. To detect PSGs in either P. euphratica or P. trichocarpa lineage, the lineage was specified in turn as the foreground branch. We then used the optimized branch-site model [55] in which likelihood ratio test P- values were computed, assuming that the null distribution was a 50:50 mixture of a χ 2 -distribution with one degree of freedom and a point mass at zero. To minimize the false discovery rate, we manually filtered all PSGs with potential errors in their alignments. Transcriptome sequencing and analysis Total RNAs were extracted and strand-specific RNA-seq libraries were generated from samples using a cetyl trimethylammonium bromide procedure [56] for transcriptome sequencing. The analysis was conducted on pooled samples of roots, leaves, flower buds, flowers, xylem and phloem from two mature male P. euphratica trees and one mature female tree from the Talim Basin desert, Xinjiang, on control samples and also on salt-stressed samples (200 mM NaCl for 6, 12, 24 and 48 h) generated from the same calluses used in genome sequencing. RNA-seq libraries were sequenced on an Illumina Genome Analyzer platform. In addition, salt-stressed leaves and roots were collected and RNA samples were isolated for Illumina short-read sequencing. Three independent biological replicate samples were examined. The resulting reads were aligned to the P. euphratica genome sequences using TopHat [48] . After alignment, the count of mapped reads from each sample was derived and normalized to fragments per kilobase of exon per million fragments mapped for each predicted transcript using the Cufflinks [49] package. DEGs were identified using the programme Cuffdiff in the Cufflinks package. We had tried to induce the calluses from P. trichocarpa , but they grew too slowly. We therefore sequenced transcriptomes of P. tomentosa calluses that had been subjected to salt-stress treatment (200 mM NaCl for 0, 6, 12, 24 and 48 h) and identified DEGs in this salt-sensitive species. In addition to the analysis as described for P. euphratica , we further assembled and annotated all reads from P. tomentosa using Trinity [57] package ( Supplementary Methods ). We used the InParanoid [58] software to identify 1:1 orthologues between P. euphratica and P. tomentosa , and aligned the coding sequences of the orthologues using Threaded Blockset Aligner [59] to extract perfectly aligned consensus blocks. Finally, we counted the reads aligned to the consensus blocks for each sample and performed edgeR [60] in R package to identify DEGs. Accession codes : The whole-genome shotgun project has been deposited in DDBJ/EMBL/GenBank nucleotide core database under the accession code AOFL00000000 . The version described in this paper is the first version, AOFL01000000 . All short-read data have been deposited in the Sequence Read Archive (SRA) under accession SRA061340 . Raw sequence data of the transcriptomes have been deposited in the SRA under accession codes SRP028829 and SRP028830 . How to cite this article: Ma, T. et al. Genomic insights into salt adaptation in a desert poplar. Nat. Commun. 4:2797 doi: 10.1038/ncomms3797 (2013).